Plant diversity increases soil microbial activity and soil carbon storage Plant diversity strongly influences ecosystem functions and services, such as soil carbon storage. However, the mechanisms underlying the positive plant diversity effects on soil carbon storage are poorly understood. We explored this relationship using long-term data from a grassland biodiversity experiment (The Jena Experiment) and radiocarbon ( 14 C) modelling. Here we show that higher plant diversity increases rhizosphere carbon inputs into the microbial community resulting in both increased microbial activity and carbon storage. Increases in soil carbon were related to the enhanced accumulation of recently fixed carbon in high-diversity plots, while plant diversity had less pronounced effects on the decomposition rate of existing carbon. The present study shows that elevated carbon storage at high plant diversity is a direct function of the soil microbial community, indicating that the increase in carbon storage is mainly limited by the integration of new carbon into soil and less by the decomposition of existing soil carbon. Climate and land use change can cause alterations in biodiversity [1] , [2] with significant consequences for ecosystem functions and services [3] . Quantifying the impact of biodiversity loss on ecosystem services requires long-term investigations in replicated experimental systems [4] , [5] , [6] . This is especially true for soil carbon storage as changes in stocks are slow [7] , the spatial heterogeneity is large [8] and the involved processes are complex [9] , [10] . Soils store the vast majority of terrestrial carbon [11] , and increased soil carbon storage may counteract the increase in atmospheric carbon dioxide. Traditional explanatory theories focus on the recalcitrance of less-reactive compounds and physical protection as controls of soil carbon stocks, while more recent theories highlight the importance of soil microorganisms for the persistence of soil organic matter. With respect to microbial regulation, emerging theories focus on either: spatial factors, which constrain the accessibility of substrates to decomposer organisms; or microbial carbon re-cycling and the consequent microbial production of soil organic matter through microbially derived products [9] , [10] , [12] , [13] , [14] , [15] . In general, the amount of carbon stored in soil represents the balance between plant shoot and root litter production, root exudates and their microbial decomposition [16] . The observed increase in carbon storage with plant diversity [17] therefore either reflects higher primary production [18] , [19] or longer persistence of plant-derived organic materials due to slower decomposition [10] , [16] . Increased plant residue inputs also provide more substrate for soil microorganisms, resulting in a more active and more abundant microbial community [20] . However, there have been different mechanisms proposed to explain how the microbial community affects soil carbon. Higher amounts of plant residue inputs might either accelerate decomposition and reduce carbon storage through decreased metabolic efficiency (microbial carbon use efficiency [21] ) or enhance decomposition of existing soil carbon (positive priming effect [22] ). Alternatively or in parallel, higher amounts of plant residue inputs could enhance carbon storage through increased microbial necromass accumulation over time [23] . Therefore, although soil carbon storage increased with plant diversity in a number of long-term grassland experiments [24] , [25] , the underlying mechanisms are yet to be understood. Here we analysed the comprehensive data collected over 9 years from The Jena Experiment, a grassland biodiversity experiment manipulating plant species and plant functional group richness [26] . Differences in plant carbon input between treatments likely originate from differences in root exudates and dead roots, as the plots were mown twice a year and aboveground plant biomass was removed as is typical for Central European hay meadows. We applied path analysis to identify the relationships between explanatory variables affecting soil carbon storage. Furthermore, to determine whether soil carbon accumulation resulted from increased root-derived carbon inputs or reduced decomposition, we modelled the carbon flow in the system using observations of soil carbon stocks and radiocarbon ( 14 C) in soil organic matter (SOM) as a double constraint [27] . The combined results of path analysis and soil carbon modelling suggest a unique cause for enhanced carbon storage with plant diversity in our experimental plots. Although both approaches are based on data from the top, biologically most active soil layer (0–5 cm), we were able to generalize the proposed mechanism of plant diversity effects on soil carbon storage to deeper soil layers (0–30 cm). Effects of plant diversity on soil organic carbon changes In 2011, 9 years after the establishment of The Jena Experiment, soil carbon concentration in the topsoil layer (0–5 cm, averaged across all diversity treatments) had increased by 27% to 4.74±0.28 g kg −1 (mean±s.e.m.). An increase in SOM was expected because the experiment had been established on a ploughed arable field turned into permanent grassland. The increase in soil carbon concentration was highly correlated with sown plant species richness ( P <0.001, Fig. 1 ). The presence of legumes negatively affected soil carbon concentration ( P =0.040, Fig. 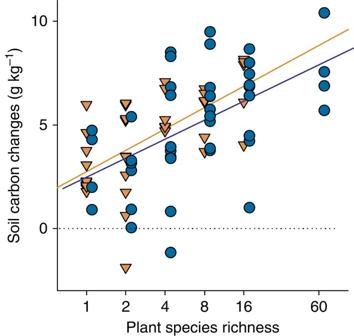Figure 1: The relationship between plant diversity and soil organic carbon storage. Soil carbon changes (g kg−1) between 2002 and 2011 as affected by (log) plant species richness (F1,73=41.29,P<0.001) and the presence (orange triangles) and absence of legumes (blue circles; F1,73=4.37,P=0.040). 1 ), while other plant functional groups or their richness did not significantly influence carbon concentration ( Table 1 ; Supplementary Table 1 ). Figure 1: The relationship between plant diversity and soil organic carbon storage. Soil carbon changes (g kg −1 ) between 2002 and 2011 as affected by (log) plant species richness (F 1,73 =41.29, P <0.001) and the presence (orange triangles) and absence of legumes (blue circles; F 1,73 =4.37, P =0.040). Full size image Table 1 Results of ANOVAs on the effects of the experimental variables. 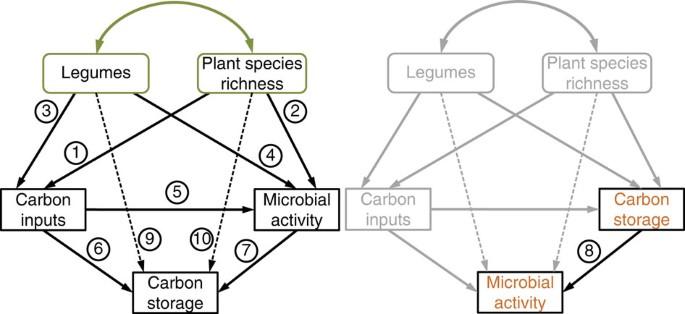Figure 2: Conceptual model on the expected causal relationships between plant diversity and soil carbon storage. The conceptual model through soil carbon inputs and soil microbial activity based on hypotheses derived from previous experiments (seeTable 2for hypotheses and references). Full size table Mechanisms of soil organic carbon storage In this strictly confirmatory approach [28] , we tested different hypotheses ( Table 2 ; Fig. 2 ), resulting in a set of different path models ( Supplementary Fig. 1 ), assessing whether the models deviate or not from the observed data structure. All individual models were tested for their adequacy in reflecting the observed data. Path analyses revealed that plant species richness had direct positive effects on root carbon inputs as well as metabolic activity of soil microorganisms, measured as basal respiration ( Fig. 3a,b ; Methods). There was no direct relationship between plant species richness or the presence of legumes and soil carbon storage, showing that fine root carbon inputs and microbial activity are the main drivers explaining the positive effect of plant diversity on soil carbon storage. Low root biomass on plots with legumes [29] may have caused the negative effect of legumes on microbial activity [20] via reduced carbon inputs. Importantly, the increased soil carbon storage was only directly related to higher microbial activity. This potential chain of causality was the best model that adequately explained the data ( Supplementary Table 2 ; Supplementary Notes 1–4 ), also when soil carbon sequestration was set up in a path model as a time series ( Supplementary Fig. 2 ), which increased the likelihood of the model. Table 2 Potential relations between the considered variables. Full size table Figure 2: Conceptual model on the expected causal relationships between plant diversity and soil carbon storage. The conceptual model through soil carbon inputs and soil microbial activity based on hypotheses derived from previous experiments (see Table 2 for hypotheses and references). 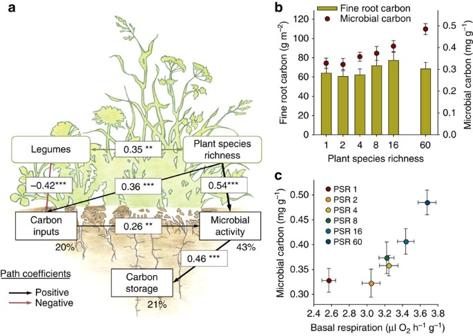Figure 3: Mechanisms of soil carbon storage. (a) Most parsimonious path model explaining the underlying mechanisms of the positive relationship between plant diversity and soil organic carbon storage (χ24=5.35,P=0.253; RMSEA=0.065 CI90 (0.000; 0.191)). Numbers next to the endogenous variables indicate their explained variance (R2). Numbers next to the arrows indicate standardized path coefficients and asterisks mark their significance: **, <0.01; or ***, <0.001. (b) Impact of (log) plant species richness on mean fine root carbon and mean soil microbial biomass. These mean values were used as specific parameters for SOM storage modelling (three-pool model) for each level of plant species richness. (c) Regression of mean metabolic activity and mean biomass of the microbial community at plant species richness (PSR) levels (R2=0.73,P=0.031). Metabolic community activity of soil microbes was measured as basal respiration and microbial community biomass was measured as microbial carbon (using chloroform fumigation analysis). Both measures are specified per g dry soil. Error bars are defined by s.e.m. RMSEA, residual mean square error of approximation. Full size image Figure 3: Mechanisms of soil carbon storage. ( a ) Most parsimonious path model explaining the underlying mechanisms of the positive relationship between plant diversity and soil organic carbon storage ( χ 2 4 =5.35, P =0.253; RMSEA=0.065 CI90 (0.000; 0.191)). Numbers next to the endogenous variables indicate their explained variance ( R 2 ). Numbers next to the arrows indicate standardized path coefficients and asterisks mark their significance: **, <0.01; or ***, <0.001. ( b ) Impact of (log) plant species richness on mean fine root carbon and mean soil microbial biomass. These mean values were used as specific parameters for SOM storage modelling (three-pool model) for each level of plant species richness. ( c ) Regression of mean metabolic activity and mean biomass of the microbial community at plant species richness (PSR) levels ( R 2 =0.73, P =0.031). Metabolic community activity of soil microbes was measured as basal respiration and microbial community biomass was measured as microbial carbon (using chloroform fumigation analysis). Both measures are specified per g dry soil. Error bars are defined by s.e.m. RMSEA, residual mean square error of approximation. Full size image Dynamics of soil organic carbon Radiocarbon-based modelling of SOM storage (Methods) suggested that the increased carbon storage in plots with higher plant species richness was mainly due to the accumulation of ‘new’ carbon ( Fig. 4a ). Furthermore, the sequestration of ‘new’ carbon and the loss of existing ‘old’ carbon (positive priming) were positively correlated ( R 2 =0.863, P =0.007, Fig. 4b ) and depended on plant species richness. High-diversity plots (richness levels 8, 16 and 60) accumulated 21.8% more carbon compared with low-diversity plots (richness levels 1, 2 and 4). At the same time, high-diversity plots primed on average only 9.6% of ‘old’ carbon. Interestingly, carbon losses were mainly observed in the fast-cycling carbon ( Fig. 4c ), whereas in the more sustainable slow-cycling carbon these losses were reduced at higher plant diversity, and more ‘new’ carbon was stored in the slow-cycling carbon ( Fig. 4d ). An explanation for these opposite patterns is the transfer or processing rate (conversion efficiency, Methods) of carbon from fast- to slow-cycling carbon, which is—in accordance with our path model—proportional to soil microbial biomass and activity ( Fig. 3c ). Consequently, the slow-cycling carbon (turnover time=47.7 years, Supplementary Table 3 ) dominates the longer-term dynamics of the total stock, whereas priming and other effects of the fast-cycling carbon (turnover time=4.0 years) become less important over longer time scales. 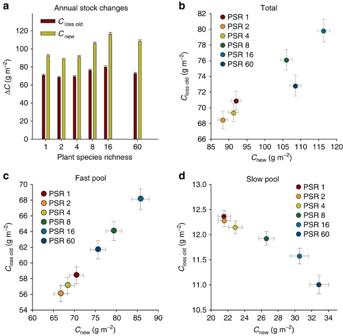Figure 4: Sequestration of new and loss of old soil organic carbon at The Jena Experiment. Effect of plant species richness (PSR) on (a) mean annual loss of old carbon (Closs old) and gain of new carbon (Cnew). Relation of new carbon sequestered and the loss of old carbon of the (b) total stock, (c) fast pool and (d) slow pool. Calculations are based on the pool model and the isotopic mass balance (Methods). Error bars are given as s.e.m. Figure 4: Sequestration of new and loss of old soil organic carbon at The Jena Experiment. Effect of plant species richness (PSR) on ( a ) mean annual loss of old carbon ( C loss old ) and gain of new carbon ( C new ). Relation of new carbon sequestered and the loss of old carbon of the ( b ) total stock, ( c ) fast pool and ( d ) slow pool. Calculations are based on the pool model and the isotopic mass balance (Methods). Error bars are given as s.e.m. Full size image The results reported in this study indicate that storage of soil carbon is governed by the metabolic activity of soil microbes, which is mediated by plant diversity via higher root inputs and other yet unidentified mechanisms, as suggested by the direct relation in the path model ( Fig. 3a ). A number of processes influence microbial activity: First, a denser vegetation in highly diverse plant communities reduces evaporation from the topsoil, which in turn promotes higher soil microbial activity and growth [30] . Second, soil carbon storage is linked to root inputs [31] , [32] including root exudation, which is known to change the activity and composition of the microbial community [33] . Indeed, carbon uptake in rhizospheric microorganisms at high plant diversity was increased compared with low plant diversity ( Fig. 5 ) as indicated by a complementary 13 CO 2 labelling experiment in the Ecotron facility in Montpellier (Methods). This showed higher microbial label uptake was most likely attributed to higher levels of root exudation with increasing plant diversity, as the soil microbial community was sampled immediately after a 3-week label application and the label enrichment in roots and root sugars was not affected by diversity (data not shown). Third, increasing diversity of soil microbial communities increases microbial respiration [34] . In fact, bacterial and fungal diversity increased with higher plant species richness in The Jena Experiment ( Table 1 ; Fig. 6 ). And finally, a shift in the metabolic activity of soil microorganisms towards anabolic activity with plant diversity resulting in increased necromass accumulation over time [23] , indicated by slightly but significantly more microbial carbon per unit root carbon in high-diversity plots ( R 2 =0.06, P =0.025). 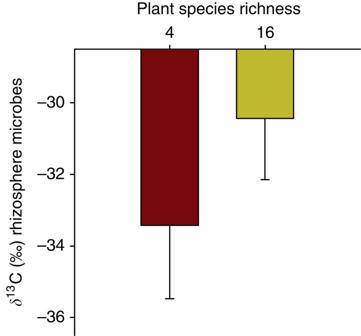Figure 5: Enrichment of root associated microorganisms in long-term13C-labelling experiment. Influence of plant species richness on the label uptake into PLFAs of the root associated microbial community (F1,9=6.99,P=0.027) studied in a 3-week labelling experiment under fully controlled conditions (ECOTRON facilities, Montpellier, France51). Error bars are given as s.e.m. Figure 5: Enrichment of root associated microorganisms in long-term 13 C-labelling experiment. Influence of plant species richness on the label uptake into PLFAs of the root associated microbial community (F 1,9 =6.99, P =0.027) studied in a 3-week labelling experiment under fully controlled conditions (ECOTRON facilities, Montpellier, France [51] ). Error bars are given as s.e.m. 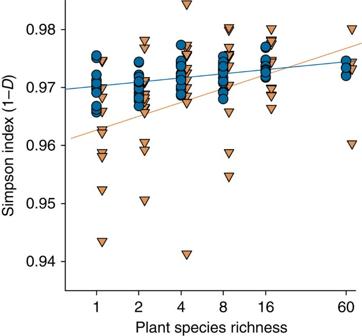Figure 6: Genetic diversity of the soil microbial community. Terminal-restriction fragment length polymorphism (TRFLP) separately analysed for fungal (orange triangles) and bacterial communities (blue circles) as affected by plant species richness (Table 1). Full size image Figure 6: Genetic diversity of the soil microbial community. Terminal-restriction fragment length polymorphism (TRFLP) separately analysed for fungal (orange triangles) and bacterial communities (blue circles) as affected by plant species richness ( Table 1 ). Full size image The missing direct path from legumes to microbial activity indicates minor importance of improvement of soil nitrogen status (measured as changes in 15 N of bulk soil, Table 1 ) for soil microbial activity, and thus for carbon storage. This was partly unexpected as legumes have been reported to increase the availability of nitrogen in soils [35] , [36] and are therefore suggested to increase plant biomass production (above and below ground) [24] , resulting in increased metabolic activity of soil microorganisms [37] . However, the presence of legumes did not increase root biomass production and the metabolic activity of soil microorganisms in The Jena Experiment [20] , [38] . Although the increase in total nitrogen content was highly correlated with the increase in soil organic carbon ( R 2 =0.79, P <0.001), the lower root biomass on legume plots [29] likely caused the negative legume effect on soil carbon storage. However, the legume effect might be most pronounced in the topsoil as it was not significant when considering the top 30 cm of the soil ( Table 1 ). In contrast, the positive plant diversity effect on soil carbon storage ( Table 1 ), root biomass [39] and soil microbial biomass [40] was also found for deeper soil layers in The Jena Experiment. Despite the consistency of the plant diversity effect, it may be strongest in the topsoil and decrease with soil depth [25] , [39] , which may be due to the fact that root carbon inputs [24] , [39] and microbial activity [41] decrease with soil depth. Therefore, the mechanism proposed for the topsoil is very likely to also be relevant for deeper soil layers, but the decreased biological activity at the deeper soil layers has to be taken into account. Moreover, other mechanisms such as spatial separation from decomposers [9] , [12] might become more important with soil depth. The positive plant diversity effect on carbon storage is driven by root carbon inputs, but mediated by the soil microbial community. Longer term, we expect this link to become even more important through both an increase of the positive plant diversity effect on plant (root) biomass production [6] , [39] and an increased microbial contribution to soil carbon storage by elevated soil microbial activity [20] . Both mechanisms in concert might be responsible for an increase of the plant diversity effect on carbon storage, as indicated by the time series path model ( Supplementary Fig. 2 ). In summary, higher levels of carbon inputs to the soil and more favourable microclimatic conditions linked to more diverse plant communities result in more active, more abundant and more diverse soil microbial communities. Microbial activity increases the turnover rates of root litter and exudates as indicated by increased microbial respiration. Thus, microbial products associated with increased microbial respiration such as microbial necromass end up in slow-cycling SOM pools in the form of reduced organic material [10] , [14] . The importance of microbial residues for soil carbon storage is suggested to even increase over time [23] . Thus, in line with the recent debate [42] , [43] , [44] , our findings challenge previous views underestimating or even negating the influence of size and activity of soil microorganisms on soil carbon storage. Our data from long-term field experiments emphasize the importance of plant diversity and its effects on soil microorganisms for ecosystem carbon storage. Although we cannot rule out that the proposed mechanisms are particularly pronounced at the field site of The Jena Experiment, the underlying relationships between plant diversity and soil carbon storage [17] , [24] , soil microbial biomass and activity [37] , [45] , [46] , and root biomass [24] , [47] have been reported in several independent experimental settings providing some evidence that the proposed links are of general significance. This leads us to reconsider the role of soil microorganisms as sources rather than sinks for slow-cycling organic matter. Thus, our results suggest that the activity and composition of soil microbial communities can serve as a proxy for carbon transfer into sustainable slow-cycling forms of soil carbon, and that plant diversity and associated soil microbial communities can significantly contribute to sequestration of atmospheric carbon dioxide. Study site of The Jena Experiment Our study was carried out as a part of The Jena Experiment, a large-scale grassland diversity experiment [26] . The experiment is located on the floodplain of the Saale River near the city of Jena (Thuringia, Germany; 50°57′ N, 11°35′ E). The soil of the field site is classified as Eutric Fluvisol [48] . In spring 2002, 82 experimental grassland plots of 20 × 20 m were established. One monoculture plot was abandoned due to poor establishment, making the total number of plots 81 instead of the 82 originally planned. Plots are arranged in four blocks to account for changes in abiotic factors with distance from the river. Soil texture in the upper soil ranges from sandy loam to silty clay with increasing distance from the river. Sand content declines from 40% near the river to 7% at the furthest plot, while silt content increases from 44 to 69%, respectively. The clay content ranges from 16 to 24%, but is not related to distance from the river. For the 40 years before establishing the experiment, the field site was a cultivated field with mineral fertilizer input. The initial physico-chemical properties, such as pH (7.1–8.4), soil organic carbon (5–33 g C kg −1 ), and soil nitrogen concentrations (1.0–2.7 g N kg −1 ), varied across the field site and are considered in the block design of The Jena Experiment [26] . The plots differed in both the number of plant species (1, 2, 4, 8, 16 and 60 species), randomly chosen from a common pool of 60 plant species, and the number of plant functional groups, that is, grasses, legumes, small herbs and tall herbs, which were classified into four functional groups based on morphological, phenological and physiological traits; for details see ref. 26 . Experimental communities are weeded manually twice a year to maintain the levels of diversity and mown twice yearly in June and September as is typical for hay meadows in Central Europe. Sampling and laboratory analyses Data included in this paper originated from soil samples taken at a depth of 0–5 cm, where biological activity is at a maximum. Fine root biomass in some cases had to be extrapolated to obtain estimates for the topsoil (0–5 cm), as not all sampling campaigns were set up for stratified sampling (see below). Soil organic carbon . Soil sampling was performed before sowing in April 2002 and was repeated in April in the years 2004, 2006, 2008 and 2011, as described in more detail in ref. 25 . In short, three soil samples were taken per plot (4.8 cm in diameter, 0–30 cm deep) using a split tube sampler (Eijkelkamp Agrisearch Equipment, Giesbeek, the Netherlands). In the year 2002, a total of five soil samples were taken per plot. The soil was dried, sieved (2 mm mesh) and milled (4 min, frequency 30 s −1 ). Total carbon of ground samples was determined by an elemental analyser after combustion at 1,150 °C (Elementaranalysator vario Max CN, Elementar Analysensysteme GmbH, Hanau, Germany). Inorganic carbon concentration was measured by elemental analysis after removing organic carbon for 16 h at 450 °C in a muffle furnace by oxidation. Organic carbon concentration was calculated from the difference between total and inorganic carbon concentrations. Carbon stocks were calculated as the product of bulk soil density and its concentration of carbon [8] . In order to exclude physical aspects of bulk density (for example, inter-annual differences caused by degree of winter freezing), statistical analyses were done with carbon concentrations (g kg −1 ) and stocks were estimated using the mean of bulk soil density across all years. Periodic sampling of other data used in this study did not always occur over the same time interval (annual: microbial activity, biannual: soil and root sampling). Thus, the mean of the other variables (basal respiration fine root carbon input) was calculated referring to each biannual soil carbon sampling campaigns. Fine root standing biomass: root standing biomass was sampled in 2003, 2004, 2006 and 2008, and separated in fine and coarse roots based on root diameter (fine roots ≤2 mm; coarse roots >2 mm). Roots were calculated as grams dry mass per square meter. In the first three sampling campaigns, fine roots were determined to a depth of 30 cm. In 2008, stratified sampling was carried out with a finer resolution of 5 cm increments. On the basis of the fine root ratio of the topsoil (0–5 cm) and entire sampling depth (0–30 cm) in 2008, fine root standing biomass in the topsoil was estimated for each prior sampling year. The carbon content of fine roots was determined using root material from ingrowth cores sampled in 2004 (ref. 29 ). Fine root biomass comprised on average 80.9% (±16.8 s.d.) of the total root biomass and was highly correlated to the total root biomass ( R 2 =0.66, P <0.001). Basal respiration . It was measured annually from 2003 to 2011, except in 2005. Five soil samples per plot were taken to a depth of 5 cm, pooled and stored at 5 °C. The samples were homogenized, sieved (2 mm) to remove larger roots, animals and stones, and adjusted to a gravimetric soil water content of 25%. Basal respiration was measured using an O 2 microcompensation apparatus [49] . The microbial respiratory response was measured at hourly intervals for 24 h at 22 °C. Basal respiration (μl O 2 h −1 per g soil dry mass) was determined without the addition of substrate and measured as the mean of the O 2 consumption rates 14–24 h after the start of the measurements (for details see ref. 20 ). Radiocarbon and soil nitrogen isotope ratios . Radiocarbon concentrations ( 14 C) were measured in soil samples of the years 2002 and 2011 as described in detail by Tefs and Gleixner [50] . Briefly, after decalcification with HCl and graphite production, the 14 C content of the samples was measured with accelerator mass spectroscopy (3 MV Tandetron 4130 AMS, High Voltage Engineering Europa, Amersfoort, The Netherlands). Soil nitrogen isotope ratios ( δ 15 N) were measured from 50 mg of dried ground soil with an elemental analyser coupled to an isotope-ratio mass spectrometer (EA-IRMS; Delta C prototype IRMS, Finnigan MAT). Root exudation . Within the experimental setup of The Jena Experiment it is not possible to determine the effects of plant diversity on the amount of root exudation. Therefore, we took advantage of the Ecotron facility in Montpellier (France) to overcome this limitation. Twelve monoliths (2.0 m in depth and 1.6 m in diameter) were excavated from the field site of The Jena Experiment and installed in the macrocosms in the Ecotron in spring 2012. These 12 monoliths reflected the diversity gradient of The Jena Experiment on a smaller scale [51] . Monoliths with high (16 plant species) and low plant diversity (4 plant species) were labelled with 13 CO 2 for 4 weeks. We analysed root exudation and the turnover of the exudates by root associated microbes using the phospholipid fatty acid (PLFA) method [52] , [53] . Particular specific monounsaturated fatty acids such as PLFA 16:1ω5, 16:1ω7, 17:1ω8 and 18:1ω7 were shown to be highly enriched by root-derived organic carbon in label experiments [54] , [55] . We measured the concentration and enrichment in δ 13 C of these PLFA markers in the Ecotron to assess the effect of plant diversity on root exudation and the incorporation of the exudates in soil microbes. Genetic diversity of soil bacteria and fungi . The genetic diversity of soil microbial communities was determined using terminal-restriction fragment length polymorphism. Briefly, total nucleic acids were extracted from 0.25 g fresh weight of soil using the MoBio Powersoil 96 kit. Bacterial 16S rRNA genes were amplified using forward primer 63F (5′-CAGGCCTAACACATGCAAGTC-3′; ref. 56 ), fluorescently labelled with 6-FAM at the 5′ end, and reverse primer 519r (5′-GTATTACCGCGGCTGCTG-3′; ref. 57 ). For fungi, we used the primer pair ITS1F (5′-CTTGGTCATTTAGAGGAAGTAA-3′) [58] and ITS4 (5′-TCCTCCGCTTATTGATATGC-3′; ref. 59 ), spanning the ITS1 and ITS2 regions. Amplicons were purified by gel filtration using Sephadex G50 (Sigma-Aldrich, Gillingham, UK) before digestion with restriction endonucleases Msp 1 (CCGG) and Taq 1 (TCGA; Promega, Southampton, UK) for bacteria and fungi, respectively. A 3730 DNA analyser (Applied Biosystems, CA, USA) was used for fragment analysis, before binning of individual terminal-restriction fragments using Genemarker software (SoftGenetics, PA, USA). The relative abundance of individual terminal-restriction fragments was calculated by dividing the intensity of each fragment by the total intensity of all fragments before calculation of Simpson’s diversity index. Statistical analyses of main effects of plant diversity The Jena Experiment is based on a factorial design with different combinations of sown plant species richness and number of functional groups. To assess for the design variables, analyses of variance with sequential sum of squares (type I SS) were applied using R [60] . The ‘block effect’, mainly accounting for differences in soil texture among the blocks [26] , was included as random factor and fitted first, followed by plant species richness and functional groups. Finally, the presence of each plant functional group (legumes, grasses, small herbs and tall herbs) was included into the model in a series of alternative models. Path analysis We applied path analyses (maximum likelihood) [28] to explore the potentially causal relationships between plant diversity and community composition and soil carbon storage using the lavaan package in R [61] . Depending on the results of the analysis of variance approach, all variables with significant effect on changes of soil carbon content were included as exogenous (predictor) variables. As variables potentially mediating plant community effects we included fine root carbon as measure of carbon input [31] , [32] and basal respiration as measure of microbial metabolic activity [20] , [34] , [37] . We tested four different ways how plant diversity can affect carbon storage: due to carbon input from roots, due to microbial activity, due to both root inputs as well as microbial activity, or directly via plant diversity, indicating that other mechanisms than root carbon input and microbial activity underlie the plant diversity effect. Each of the four storage ways comprised a set of models ( Supplementary Fig. 1 ), differing in the relations from plant diversity to basal respiration and fine root carbon to basal respiration. For all models, the adequacy of the hypothesized structural relationships and the data was verified using χ 2 -tests and the residual mean square error of approximation. To test whether carbon storage is a function of the microbial activity or vice versa, we tested all models twice, first with the path from basal respiration towards soil carbon content, as ‘sink models’ (as described above, Supplementary Note 1 ) and second with a path from soil carbon content towards basal respiration as ‘source models’ ( Supplementary Note 2 ). In the final step, we identified the minimal adequate (most parsimonious) model based on the Bayes Information Criterion. Therefore, all adequate models were compared ( Supplementary Note 3 ), including nonsignificant pathways and when only significant pathways are contained. Eisenhauer et al. [20] and Ravenek et al. [39] showed that plant species richness was not closely linked to basal respiration and root standing biomass in the first years of the experiment; therefore, we did not use data from the first 2 years in the present analyses. Missing values were replaced by the mean. All variables were standardized to (0, 1). The total sample size was N =81. Three-pool 14 C model with serial structure To describe soil organic carbon dynamics in The Jena Experiment, we implemented a dynamic model of the form where C f , C s and C p represent carbon storage in the fast, slow and passive pool, respectively. I represents the total amount of carbon input to the first 5 cm of the soil, and k 1 , k 2 and k 3 represent first-order decomposition rates for the fast, slow and passive pools, respectively. The transfer coefficients α 2,1 and α 3,2 represent the proportion of the decomposed carbon from each pool that is transferred to a slower cycling pool [62] , [63] . One particular aspect of this model, suggested from the path analysis, is that we represent the effects of the microbial community on decomposition as a control on the transfer rate. That is, we assume where MB is the microbial biomass and f is a scaling factor. Notice that we do not represent the microbial biomass as an additional pool in our dynamical system because it leads to unrealistic nonlinear behaviour [64] not supported by our own observations. To account for radiocarbon dynamics, we implemented a model similar to equation (1) representing each pool as a fraction of radiocarbon with respect to an internationally agreed standard [27] , [63] . The model has similar form as equation (1) with an additional term accounting for radioactive decay. The model was implemented in the R environment for computing using the SoilR package [65] . The passive pool is mainly needed to account for the low 14 C values in the bulk soil organic matter. As described by other authors [66] , such low 14 C values are common for arable fields in Europe. On the basis of our findings in the path analysis, we implemented a measure of soil microbial community activity (basal respiration) as a proxy for the transfer between the fast and slow carbon pool. Unfortunately, no data on basal respiration were available for arable control plots, which would have been needed for the spin up (please see section ‘Spin up and parameter estimation for the spin up’). Thus, we took advantage of the microbial biomass (based on the chloroform fumigation extraction analysis [67] ) instead. Basal respiration and microbial biomass were highly correlated ( Fig. 3c ). For each level of plant species richness, we applied a model with the level specific parameter estimation ( Table 1 ; Fig. 3b ). However, we could neither evaluate the real carbon input (carbon of standing fine root biomass and root exudates, root tips and so on) nor the extent of the transfer coefficient. Thus, we applied a set of different models for each level of plant diversity, modified in the carbon input and transfer coefficient. Implementing the transfer coefficient between the fast and the slow pool depending on soil microbial biomass resulted in good agreement between model predictions and measured data ( Table 3 ; Supplementary Table 3 ; and Supplementary Fig. 3 ). Table 3 Variations of soil carbon properties and their drivers in The Jena Experiment. Full size table Calculation of new carbon accumulated and loss of old carbon: on the basis of the mass balance and the isotopic mass balance for the isotopic mass ratio (equation (3)), we calculated the yearly (a) amount of new carbon sequestrated ( C new ) and loss of the old carbon ( C loss old ). Spin up and parameter estimation for the spin up . The objective of the spin up simulations is to match the carbon stocks and 14 C data for the pre-experimental conditions. We let the spin up simulations run for 10,000 years to assure the modelled pre-experimental conditions are in equilibrium. As there are no comparable data for fine root biomass on the arable control plots, we used the mean fine root carbon of all experimental plots from of all fine root sampling campaigns (mean=149.77 g m −2 , s.d.=98.05). Due to ploughing of the soil before the implementation of the experimental plots, a homogeneous distribution of fine root carbon can be assumed as 25 g m −2 in each soil segment of 5 cm. In contrast, after establishment of experimental plots, the fine root biomass distribution was similar to meadows with the main amount of roots in the topsoil, strongly decreasing towards deeper depths. Thus, a fine root carbon input of 67.04 g m −2 (on average) was assumed on experimental plots. The ratio of the assumed fine root inputs between experimental plots and arable land is similar to the ratio of carbon input on meadows and arable lands reported in ref. 68 Furthermore, we applied a fine root turnover of 1.7 years on experimental grassland plots [69] . To meet the measured and the modelled data, a fine root turnover of 1.2 years for arable lands was applied. In the spin up, we set the input factor to 1.7 ( Supplementary Table 3 ), the transfer coefficient to 0.1 reflecting C mic of 0.22 ng g −1 on the arable control plots (cf. Table 1 ). This value of the transfer coefficient is within the expected range. The resulting sizes of the three pools and their ages are shown in Supplementary Table 3 . How to cite this article: Lange, M. et al. Plant diversity increases soil microbial activity and soil carbon storage. Nat. Commun. 6:6707 doi: 10.1038/ncomms7707 (2015).